Interpreting carbonate and organic carbon isotope covariance in the sedimentary record Many negative δ 13 C excursions in marine carbonates from the geological record are interpreted to record significant biogeochemical events in early Earth history. The assumption that no post-depositional processes can simultaneously alter carbonate and organic δ 13 C values towards more negative values is the cornerstone of this approach. However, the effects of post-depositional alteration on the relationship between carbonate and organic δ 13 C values have not been directly evaluated. Here we present paired carbonate and organic δ 13 C records that exhibit a coupled negative excursion resulting from multiple periods of meteoric alteration of the carbonate δ 13 C record, and consequent contributions of isotopically negative terrestrial organic matter to the sedimentary record. The possibility that carbonate and organic δ 13 C records can be simultaneously shifted towards lower δ 13 C values during periods of subaerial exposure may necessitate the reappraisal of some of the δ 13 C anomalies associated with noteworthy biogeochemical events throughout Earth history. Significant events in Earth history are often associated with major changes in the carbon isotopic composition of marine carbonates ( δ 13 C carb ) and co-occurring sedimentary organic matter ( δ 13 C org ). Globally correlatable excursions in marine δ 13 C carb records are often thought to be related to global changes in the carbon cycle, such as those induced by snowball Earth events in the Neoproterozoic [1] , [2] , [3] , the oxygenation of Earth’s atmosphere [4] , [5] , [6] , [7] , the evolution of Ediacaran metazoans [8] , [9] , as well as marine and terrestrial extinction episodes [10] , [11] , [12] , [13] , [14] . A common approach used to establish whether the variations in a δ 13 C carb record reflect changes in the isotopic composition of the ancient dissolved inorganic carbon pool is to assess the covariation between coeval carbonate and sedimentary organic carbon isotope records [15] , [16] , [17] , [18] , [19] , [20] , [21] , [22] . Classically, covariant δ 13 C carb and δ 13 C org records are interpreted as evidence that both the carbonate and organic matter were originally produced in the surface waters of the ocean, and that they have retained their original δ 13 C composition [10] , [19] , [20] , [21] , [22] , [23] , [24] , [25] , while decoupled δ 13 C carb and δ 13 C org records have been interpreted as evidence for diagenetic alteration [16] , [19] , [20] , [26] , the ‘Rothman ocean’ model [27] , or that local syn-sedimentary processes have made the δ 13 C org record noisy [8] . The application of covariance between δ 13 C carb and δ 13 C org is based upon the theoretical assumption that ‘….no secondary processes are known (or for that matter, conceivable) which always shift the isotopic composition of carbonate and organic carbon in the same direction at the same rate…’ [20] . This assumption has been widely used to establish the original nature of Precambrian and Palaeozoic δ 13 C carb records derived from shallow platform and marginal marine carbonates [10] , [15] , [16] , [19] , [20] , [22] . Consequently, the analysis of coeval δ 13 C carb and δ 13 C org values have been a fundamental approach in studies of Precambrian and Palaeozoic carbon cycling, because it is thought to distinguish geologically meaningful records of significant biogeochemical changes in Earth history from those records that have been altered by diagenesis. Since shallow marine deposits may have been periodically subaerially exposed during sea-level oscillations, it is important to address the possibility of diagenetic alteration. This is particularly important since freshwater alteration has been shown to generate negative δ 13 C carb excursions that are similar in magnitude to those observed in early Earth history [28] . Although a variety of other diagnostic tools have been employed to assess the degree of alteration, including trace element ratios [29] , [30] , cathodoluminescence [31] , [32] , as well as the relationship between δ 13 C carb and δ 18 O carb records [33] , [34] , [35] , the covariance between δ 13 C carb and δ 13 C org records is thought to prove that the system is ‘rock buffered’ and that the records have retained their initial δ 13 C values [10] , [15] , [16] , [19] , [20] , [22] . Remarkably, however, the effects of diagenesis on the relationship between carbonate and organic δ 13 C records have never been directly investigated. Here we evaluate the effects of post-depositional alteration on paired δ 13 C carb and δ 13 C org values from a core that has unequivocally been altered by freshwater and marine diagenetic processes (‘Clino’, Fig. 1 ). More than 470 paired δ 13 C measurements were conducted on this ~700-m core that was drilled into the margin of the Great Bahama Bank [36] . During the late-Pleistocene, multiple sea-level oscillations exposed the upper 120 m of the platform to the influence of meteoric waters. Ten subaerial exposure surfaces have been identified in the top 100 m of the core, each of which is proposed to have been related to a Pleistocene glacial period [37] , [38] . Evidence of both meteoric and marine diagenesis has been recorded within this 5.3 Ma record of marginal and shallow marine carbonates [39] , [40] , [41] , including the development of caliche crusts, blocky spar cements, large-scale dissolution and soil development [37] , [38] , [40] . Evidence of marine burial diagenesis includes non-depositional surfaces in the core [42] , which in some cases are associated with dolomites containing negative δ 13 C carb signatures [43] . Paired δ 13 C carb and δ 13 C org analyses in these altered sediments are strongly covariant throughout the length of the core, particularly in the Plio–Pleistocene section of the record. These results demonstrate how post-depositional processes, linked in time by subaerial exposure, have shifted the isotopic composition of carbonate and organic carbon in the same direction at the same time. 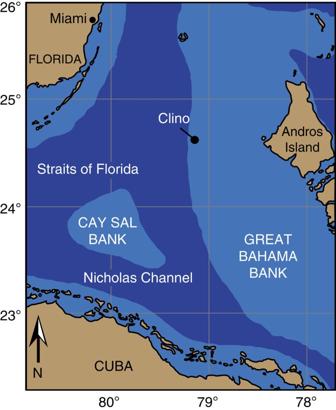Figure 1: Location of Clino core. Clino was drilled on the platform top of the Great Bahama Bank, and the water depth at the time of drilling was 7.6 m (ref.36). Figure 1: Location of Clino core. Clino was drilled on the platform top of the Great Bahama Bank, and the water depth at the time of drilling was 7.6 m (ref. 36 ). Full size image Bulk geochemical relationships from Clino The Clino core has previously been separated into three diagenetic zones based upon petrographic characteristics and δ 13 C carb and δ 18 O carb values [39] . Although the bulk δ 13 C carb and δ 18 O carb ( Fig. 2a , r 2 =0.44, P <0.05, n =465) and δ 13 C carb and δ 13 C org values ( Fig. 2b , r 2 =0.59, P <0.05, n =465) show statistically significant positive correlations, the relationships are variable within each of the different diagenetic environments ( Fig. 3a,b ). The δ 13 C carb and δ 13 C org data ( Supplementary Table 1 ) are considered within this framework. 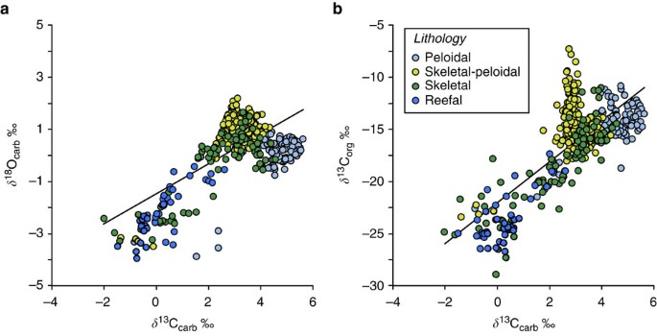Figure 2: Relationship between isotope records from the whole core subdivided by lithology. (a) Correlation betweenδ13Ccarbandδ18Ocarbvalues from the entire length of the core Clino (r2=0.44,P<0.05,n=465) subdivided by published lithological assignments37,42. (b) Relationship betweenδ13Ccarbandδ13Corgvalues from the entire length of the core Clino (r2=0.59,P<0.05,n=465) subdivided by published lithological assignments37,42. Figure 2: Relationship between isotope records from the whole core subdivided by lithology. ( a ) Correlation between δ 13 C carb and δ 18 O carb values from the entire length of the core Clino ( r 2 =0.44, P <0.05, n =465) subdivided by published lithological assignments [37] , [42] . ( b ) Relationship between δ 13 C carb and δ 13 C org values from the entire length of the core Clino ( r 2 =0.59, P <0.05, n =465) subdivided by published lithological assignments [37] , [42] . 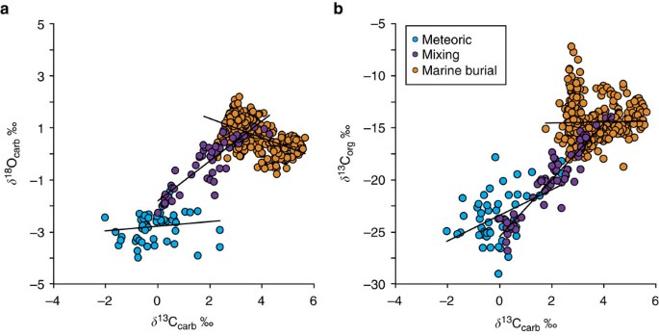Figure 3: Relationship between isotope records subdivided by the diagenetic zone. (a) Correlations betweenδ13Ccarbandδ18Ocarbrecords from the diagenetic zones defined by Melimet al.(ref.39): meteoric (blue circles,r2=0.01,P>0.05,n=53), mixing (purple circles,r2=0.81,P<0.05,n=58) and marine burial (orange circles,r2=0.22,P<0.05,n=354). (b) Relationship betweenδ13Ccarbandδ13Corgvalues subdivided by diagenetic zones: meteoric (blue circles,r2=0.21,P>0.05,n=53), mixing (purple circles,r2=0.87,P<0.05,n=58) and marine burial (orange circles,r2=0.06,P>0.05,n=354). Full size image Figure 3: Relationship between isotope records subdivided by the diagenetic zone. ( a ) Correlations between δ 13 C carb and δ 18 O carb records from the diagenetic zones defined by Melim et al. (ref. 39 ): meteoric (blue circles, r 2 =0.01, P >0.05, n =53), mixing (purple circles, r 2 =0.81, P <0.05, n =58) and marine burial (orange circles, r 2 =0.22, P <0.05, n =354). ( b ) Relationship between δ 13 C carb and δ 13 C org values subdivided by diagenetic zones: meteoric (blue circles, r 2 =0.21, P >0.05, n =53), mixing (purple circles, r 2 =0.87, P <0.05, n =58) and marine burial (orange circles, r 2 =0.06, P >0.05, n =354). Full size image Geochemical relationships within each diagenetic zone The uppermost portion of Clino (0–100 m), corresponding to the vadose and freshwater phreatic zones [35] , is characterized by large variations in the δ 13 C carb record and rather constant, but negative δ 18 O carb values. Throughout this interval there are abundant subaerial exposures ( Fig. 4 ), which have more negative δ 13 C carb values (but constant and negative δ 18 O carb ) and high concentrations of trace metals such as Fe and Mn [37] . The δ 13 C carb and δ 18 O carb values are not statistically significantly correlated ( Fig. 3a ), the concentration of total organic carbon (TOC) is <0.1% ( Fig. 4 ) and there is no statistically significant correlation between the δ 13 C carb and δ 13 C org within the meteoric zone ( r 2 =0.21, P >0.05, n =53, Fig. 3b ). Between 100 and 200 m, there is a transition from negative to positive δ 13 C carb and δ 18 O carb values (the ‘mixing zone’ [35] ) ( Fig. 4 ). This portion of the core exhibits a very strong positive correlation between the δ 13 C carb and δ 18 O carb values ( Fig. 3a ), as well as between the δ 13 C carb and δ 13 C org values ( r 2 =0.87, P <0.05, n =58, Fig. 3b ). Below the ‘mixing zone’ there is a region in which there are relatively positive δ 13 C carb and δ 18 O carb values, an area interpreted as having been affected only by marine diagenesis [39] . The marine burial zone shows no statistically significant relationship between the δ 13 C carb and δ 18 O carb ( Fig. 3a ) or between δ 13 C carb and δ 13 C org values ( r 2 =0.06, P >0.05, n =354, Fig. 3b ). The concentration of TOC increases through the ‘mixing zone’ and is an order of magnitude higher in the marine burial zone reaching values up to 1.2% ( Fig. 4 ). 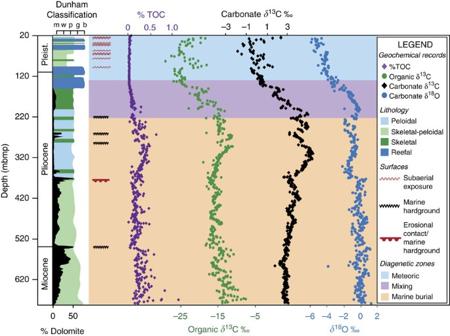Figure 4: Geochemical records and lithostratigraphy of Clino. Total organic carbon (TOC) content, carbonateδ13C values, organicδ13C values and carbonateδ18O values (n=465 for each record) produced by this study from the Neogene carbonates in the core Clino. The data used to construct the simplified stratigraphic column presented in this figure were obtained from Kenteret al.(ref.42) and Kievman (ref.37). Diagenetic zones (‘meteoric’, ‘mixing’ and ‘marine burial’) were defined by published interpretations of both petrographic40and isotopic constraints35. The record of percent dolomite was determined by X-ray diffractometry39. Figure 4: Geochemical records and lithostratigraphy of Clino. Total organic carbon (TOC) content, carbonate δ 13 C values, organic δ 13 C values and carbonate δ 18 O values ( n =465 for each record) produced by this study from the Neogene carbonates in the core Clino. The data used to construct the simplified stratigraphic column presented in this figure were obtained from Kenter et al. (ref. 42 ) and Kievman (ref. 37 ). Diagenetic zones (‘meteoric’, ‘mixing’ and ‘marine burial’) were defined by published interpretations of both petrographic [40] and isotopic constraints [35] . The record of percent dolomite was determined by X-ray diffractometry [39] . Full size image The zone of meteoric alteration in Clino has the lowest δ 13 C carb (−2 to +2‰) and δ 13 C org (−29 to −17‰) values, and no statistically significant covariance between δ 13 C carb and δ 13 C org ( Fig. 3b ). Both the δ 13 C carb and δ 13 C org values are significantly lower than those reported for modern shallow marine sediments from Great Bahama Bank, which average +4.5 and −12‰, respectively [44] , [45] . We suggest that these low δ 13 C carb values arise from the oxidation of organic matter, which imparts a low δ 13 C value to the dissolved inorganic carbon, along with cementation, mineralogical stabilization and recrystallization of the carbonate [33] , [39] . Concurrently, δ 13 C org values became more negative as the labile marine organic matter was oxidized, and additional organic material was contributed from terrestrial C 3 plants and freshwater algae, which colonized the newly exposed platform top. Multiple subaerial exposures of the platform top during the Pleistocene have superimposed the effects of such diagenetic processes on the carbonates and organic matter preserved in Clino, and as a result, the records currently observed are the cumulative product of these post-depositional changes. Although preferential degradation of labile organic compounds can cause the δ 13 C org value of the residual organic carbon to become more positive [46] , in the majority of cases degradation has been shown to produce residual organic carbon with more negative δ 13 C org values [47] , [48] , [49] . However, these processes can only produce changes of up to 4–5‰ in the δ 13 C org record [46] , [48] , [49] , [50] , [51] , and since the lowest δ 13 C org value of sedimentary organic matter from the platform top is −17‰ (ref. 45 ), diagenetic reactions alone could not have produced the δ 13 C org values of −29‰ observed in the upper 200 m of Clino. Consequently, a source of organic carbon with a δ 13 C org value lower than −22‰ is required to produce the δ 13 C org values observed in the top 100 m of the core. Such a source is likely to be terrestrial C 3 plant matter, such as mangroves and freshwater algae, which have δ 13 C org values ranging from −20 to −32‰ (ref. 52 ). Evidence of terrestrial plant contribution is provided by root casts observed in the subaerial exposure surfaces [37] ( Supplementary Figs 1 and 2 ). In addition, terrestrial organic matter is known to be preferentially preserved through time, especially in oxidizing settings where marine organic compounds have been found to be degraded twice as fast as terrestrial soil-derived organic compounds [53] . We suggest that these post-depositional processes may account for the low concentration of organic carbon (<0.2%), the negative δ 13 C org values ( Fig. 2 ) and the increase in the proportion of low-magnesium calcite [40] in the section of the core affected by meteoric diagenesis. The highest correlation between the δ 13 C carb and δ 13 C org values ( Fig. 3b ) is observed between 100 and 200 mbmp, in the section of the core associated with a strong correlation between δ 13 C carb and δ 18 O carb . The strong positive correlation between δ 13 C carb and δ 13 C org records in the ‘mixing zone’ ( Fig. 3b ) can be attributed to a gradient of post-depositional changes. The sediments and organic matter preserved closer to 100 mbmp exhibit low δ 13 C carb and δ 13 C org values, because they have been repeatedly affected by freshwater diagenetic reactions and post-depositional contributions of terrestrial organic matter, as previously described. In contrast, the δ 13 C carb and δ 13 C org values in the section of the core closer to 200 mbmp are comparatively more positive, and similar to those observed both on the modern platform top [45] as well as those preserved in the marine burial zone ( Fig. 4 ), suggesting that this section of the core has experienced fewer episodes of alteration and lower contributions, if any, of terrestrial organic carbon. The δ 13 C carb and δ 13 C org records in the marine burial diagenetic zone probably represent the least altered values within the entire core. The absence of covariance between δ 13 C carb and δ 13 C org records, and the range of δ 13 C carb and δ 13 C org values in the marine burial diagenetic zone ( Fig. 3b ) are similar to unaltered Pleistocene periplatform sediments deposited on the slope of the Great Bahama Bank [45] . Throughout the marine burial zone, there are minor variations in δ 13 C carb and δ 13 C org that represent subtle changes in the source of the sediments through time, as well as diagenetic processes. An example of the influence that a change in source can have on both the δ 13 C carb and δ 13 C org values is the synchronous change towards more positive values observed at 367 mbmp. At this depth, the background sediment type changes from a mixed peloidal-skeletal packstone with significant contributions from pelagic foraminifera, to a peloid-dominated chalky wackestone to packstone almost entirely devoid of planktic foraminifera [42] . The synchronous positive shifts in the δ 13 C carb and δ 13 C org records are consistent with increased off-bank shedding as the platform prograded towards the Straits of Florida during the Pliocene [54] , [55] . Off-bank shedding would have contributed increasingly higher proportions of platform-derived carbonates and organic matter, which are characterized by relatively higher δ 13 C carb and δ 13 C org values [45] . Minor fluctuations in the δ 13 C carb and δ 13 C org records occur at marine hardgrounds ( Fig. 4 ) [42] , and are likely associated with the oxidation of marine organic matter and the precipitation of dolomite below non-depositional surfaces [43] within the marine burial diagenetic zone. This data set clearly demonstrates how two post-depositional changes linked in time by periods of subaerial exposure, the diagenetic alteration of the carbonate and the post-depositional contribution of terrestrial organic carbon, can produce negative excursions with highly covariant δ 13 C carb and δ 13 C org records. The excursion observed in the Neogene is similar in magnitude to those observed in Palaeozoic and Precambrian deposits. Whether or not those ancient deposits were exposed to the same degree of freshwater alteration as Clino is still a matter of debate [28] . In many cases, negative δ 13 C carb excursions have been interpreted to be pristine records of global carbon cycling [15] , [19] , [20] , [21] , [56] , [57] , because sedimentological evidence of subaerial exposure was not observed [26] , [58] . However, subaerial exposure surfaces can be cryptic in the rock record, and other workers have interpreted the same geochemical changes to be diagenetic in origin [28] , [59] . If the latter is true, and multiple sources of organic carbon contributed to the sedimentary organic matter preserved in the deposit, as was recently shown to be the case for the Ediacaran Shuram Formation in Oman [60] , then the model presented here could conceivably explain covarying trends in paired δ 13 C carb and δ 13 C org records from the ancient geological record. Although higher level terrestrial plants were not present until the late Palaeozoic, the presence of terrestrial life in earlier time periods, including photosynthetic cyanobacteria, fungi and algae [61] , [62] , [63] , [64] , [65] , [66] , supports the possibility that ancient sedimentary organic carbon could have been composed of mixtures of marine and terrestrial organic carbon, in a situation analogous to the model of subaerial exposure proposed for the Neogene. In fact, the range in δ 13 C org values of Precambrian sedimentary organic matter is the largest for any time period in Earth history [67] . Although the organisms were different in the ancient geological record, processes similar to those described here could have occurred. In contradiction to the assumption that coupled negative excursions in δ 13 C carb and δ 13 C org values can only be produced by changes in the global carbon cycle, these results suggest that post-depositional processes can play an influential role in generating covariant δ 13 C carb and δ 13 C org values. Consequently, interpretations of strongly correlated δ 13 C carb and δ 13 C org values from the ancient geological record should reconsider the influence that similar post-depositional processes may have in generating some of the coupled negative excursions associated with noteworthy biogeochemical events in early Earth history. Sampling strategy Clino was sampled at roughly 1.5 m intervals to obtain at least 50 samples per diagenetic zone (meteoric zone, n =53, mixing zone, n =58 and marine burial diagenetic zone, n =354). However, major sedimentological features such as subaerial exposure surfaces and hardgrounds were avoided to preserve limited core material. Such features had been sampled in previous studies [39] , [40] , [41] , which accounts for the larger ranges in δ 13 C carb reported in those studies. For each paired carbon isotope data point, roughly a gram of bulk sediment was powdered and homogenized to provide subsamples for carbonate and organic carbon isotope analysis. Carbonate δ 13 C and δ 18 O measurements Carbonate δ 13 C and δ 18 O values were analysed via dissolution in phosphoric acid using the common acid bath method [68] . The CO 2 gas produced by the reaction of phosphoric acid and carbonate was analysed on a Finnigan MAT 251 (Thermo Fisher Scientific, Bremen, Germany). In each run of 24 samples, four standards were processed at the start of the run and two at the end, followed by a measurement of the zero enrichment. Data were then corrected for any fractionation in the reference gas during the run and for the usual isobaric interferences modified for a triple collector mass spectrometer. Data are reported relative to the Vienna Pee Dee Belemnite (VPDB) scale, defined for carbonates by the δ 13 C value of NBS-19 (1.95‰ versus Pee Dee Belemnite (PDB) [69] ). The error for these analyses is <0.1‰ as indicated by replicate analyses of internal standards. Organic δ 13 C and TOC measurements Co-occurring sedimentary organic material was separated via dissolution in 10% HCl acid overnight, followed by subsequent vacuum filtration onto glass microfiber filters (Whatman GF/C). The insoluble residue (IR) on the filter was allowed to dry for at least 48 h, or until a constant dry weight was achieved. The weights of the insoluble material were quantified by subtracting the weight of the empty filter from the weight of the dried insoluble material and filter after filtration. Samples of the insoluble material were scraped off of the filters, weighed and packed into tin capsules and loaded into a Costech ECS 4010 (Costech Analytical Technologies Inc., Valencia, CA, USA), where they were combusted. The resulting CO 2 gas transferred for isotopic measurement to a continuous flow isotope-ratio mass spectrometer (Delta V Advantage, Thermo Fisher Scientific). For every run of 36 samples, 12 internal standards were analysed to calibrate the machine and to assess the precision of the measurements. An analytic blank and 6 internal standards preceded the first sample analysis, and two standards were run for every 10 samples analysed. The reproducibility of δ 13 C values is ±0.1‰ as indicated by the s.d. of replicate analyses of internal standards of glycine ( n =54, δ 13 C value=−31.8‰ VPDB). All δ 13 C org data are reported relative to the VPDB scale, defined for organic carbon as the δ 13 C value of graphite (USGS24)=−16.05‰ versus VPDB [70] . To calculate weight percent carbon in the IR, a calibration line was established that related the peak area measured by the Delta V Advantage (Thermo Fisher Scientific) to the known weight of carbon in the internal standard, glycine. The weights of the standards were chosen to bracket the expected range of organic carbon in the samples. The s.d. of these analyses is 0.4% based upon repeated analyses of glycine ( n =54). Delta V Advantage peak area measurements for each sample was transformed to mg of organic carbon in the insoluble residue using the equation of the calibration line. Organic carbon concentration in the insoluble residue in mg was converted to TOC by the following equation: TOC=((Org C in IR (mg) × total IR weight (mg))/initial weight of the sediment (mg)) × 100 Statistical analyses Pearson’s regression analysis was used to determine the relationship between isotope records. The r 2 , P and n values are listed in the main text for each analysis conducted. How to cite this article: Oehlert, A. M. and Swart, P. K. Interpreting carbonate and organic carbon isotope covariance in the sedimentary record. Nat. Commun. 5:4672 doi: 10.1038/ncomms5672 (2014).